Site-selective photoemission from delocalized valence shells induced by molecular rotation Due to the generally delocalized nature of molecular valence orbitals, valence-shell spectroscopies do not usually allow to specifically target a selected atom in a molecule. However, in X-ray electron spectroscopy, the photoelectron momentum is large and the recoil angular momentum transferred to the molecule is larger when the photoelectron is ejected from a light atom compared with a heavy one. This confers an extreme sensitivity of the rotational excitation to the ionization site. Here we show that, indeed, the use of high-energy photons to photoionize valence-shell electrons of hydrogen chloride offers an unexpected way to decrypt the atomic composition of the molecular orbitals due to the rotational dependence of the photoionization profiles. The analysis of the site-specific rotational envelopes allows us to disentangle the effects of the two main mechanisms of rotational excitation, based on angular momentum exchange between the molecule and either the incoming photon or the emitted electron. Controlling electronic [1] and/or nuclear [2] , [3] motion in molecules using external fields represents, at the moment, the ‘holy grail’ of chemistry. More than half a century ago, the 1966 Nobel Prize winner Alfred Kastler achieved an important step towards increasing the angular momentum transfer from photons to atoms by repeated absorption/spontaneous emission cycles [4] . The active control by light of the rotational degrees of freedom in molecules is a cornerstone of modern quantum physics. In particular, the angular momentum exchange between photons and molecules is at the basis of numerous applications, such as the spatial orientation and alignment of molecules by weak [5] or strong laser fields [6] , rotational heating [7] or light-driven rotary molecular motors [8] , [9] . At the same time, a series of molecular, laser-based multi-photon experiments [10] , [11] , [12] showed that a significant degree of angular momentum transfer can be achieved by climbing up a rotational ladder. The molecular centrifuge effect [10] , [12] even allows breaking chemical bonds. In contrast to multi-photon rotational heating, the increase of angular momentum in a molecule by single-photon X-ray absorption processes can be explored as an original opportunity to achieve site selectivity in valence-shell photoionization. We studied X-ray valence photoionization of hydrogen chloride, where the valence electrons are ejected coherently from both hydrogen and chlorine sites. However, the rotational excitation of the molecule is much more efficient when the fast photoelectron is ejected from the light hydrogen atom site, and this site-selective behaviour can be observed experimentally as described below. This strongly site-dependent rotational excitation of the molecule can be achieved because the torques created by the electrons ejected from the hydrogen or from the chlorine sites differ by more than one order of magnitude. This effect allows us to unambiguously identify the site from which the electron was ejected in spite of the delocalized nature of the valence hole in the molecular cation left behind. The selectivity originates from the large torque induced by the photoelectron on the H-site, creating a very broad and shifted rotational band related to the hydrogen emission. It is, thus, possible to spectroscopically separate the H rotational band from the narrow and intense Cl rotational band. This separation allows one to monitor the molecular orbital (MO) extension at different atomic sites, and hence to map the composition of MOs. Rotational heating by X-ray valence photoionization Rotational excitation of the HCl molecule can be achieved either directly, by the absorption of an X-ray photon, or induced by the fast photoelectron ejected in the photoionization process of the 5σ valence MO. This delocalized MO, with the ionization potential I 5σ =16.3 eV for the vibrational level v=0, is a linear combination of atomic wave functions φ H and φ Cl , localized near the H and the Cl atoms, respectively, separated by the distance R . At first sight, the ionization site cannot be known because the electron cloud of the ψ 5σ MO is delocalized over both the atoms. However, this first impression is not correct, as one can see from the valence photoionization amplitude , which is the sum of the ionization amplitudes for the hydrogen b H ( k ), and for the chlorine b Cl ( k ) atoms. Here the factor e i k · R n is responsible for the momentum and the angular momentum transfer from the electron to the molecule [13] , [14] , [15] , [16] , [17] , [18] , [19] , [20] , [21] , [22] , [23] , [24] . The radius vector (lever) R n between the n th atom and the centre of gravity of the molecule is large for the light hydrogen atom, but it is very small for the heavy chlorine atom ( R Cl / R H = m H / m Cl ≈0.028). This means that the recoil angular momentum j n = R n × k transferred by the ejected electron to the molecule is much larger for hydrogen than for chlorine: for E =84 eV, where θ is the angle between k and the molecular axis. Thus, we reach the important conclusion that the photoionization-induced rotational heating of the HCl molecule is very sensitive to the ionization site. Site selectivity of the rotational excitation The rotational excitation is weak in the case when the electron is ejected from the heavy Cl atom because the recoil angular momentum is small, . In this case, the ‘HCl-wheel’ is rotated mainly due to the transfer of the photon spin to the molecule via the light polarization e (see Fig. 1 ). The spinning of HCl is much faster when the electron is emitted from the hydrogen site, in this situation the main mechanism of rotational excitation being the ejection of the photoelectron, rather than the photon-spin transfer. In the latter case, the rotation is dramatically enhanced due to the recoil experienced by the molecule during photoelectron ejection from the light H atom. The large recoil angular momentum results in a large rotational Doppler shift ω · j (refs 22 , 25 ) and in a red shift of the photoelectron line owing to the rotational recoil effect [23] j 2 (θ)/2 I ( Fig. 1 ). Here I is the moment of inertia in the lowest vibrational sub-state and ω is the angular velocity of the molecule in the ground state. 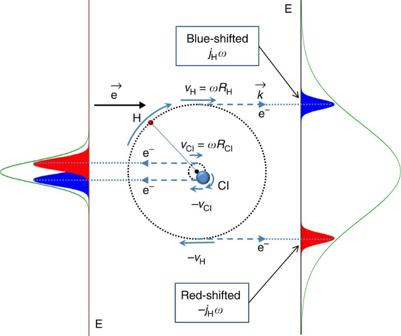Figure 1: Physical picture of the site selectivity achieved by X-ray rotational heating. The rotational heating is caused by the angular momentum transferred to the molecule by the electron ejected from the heavy Cl or the light H atoms. In the ground state, the molecule rotates with the angular velocityωdue to the finite temperature. The hydrogen and chlorine atoms have different distances from the centre of gravity, whereM=mH+mClis the total mass of the molecule. This makes the velocity of the light H atom much larger than the velocity of the heavy Cl atom:. During the rotation, the electron energy will exhibit a Doppler shift, which changes in the interval (−kωRn,+kωRn) due to the change in the anglebetweenvnand the electron momentumk. This variation of the Doppler shift results in a Doppler line broadening which is different for light (n=H) and heavy (n=Cl) atoms. Taking into account thatjn=Rn×k, we can conclude that the Doppler shiftk·vnis nothing else but the rotational Doppler shiftjn·ω, which is larger for the light atom. The X-ray polarization vectoreis parallel to the electron momentumk, while the photon propagation axis is perpendicular to the figure plane. Figure 1: Physical picture of the site selectivity achieved by X-ray rotational heating. The rotational heating is caused by the angular momentum transferred to the molecule by the electron ejected from the heavy Cl or the light H atoms. In the ground state, the molecule rotates with the angular velocity ω due to the finite temperature. The hydrogen and chlorine atoms have different distances from the centre of gravity , where M = m H + m Cl is the total mass of the molecule. This makes the velocity of the light H atom much larger than the velocity of the heavy Cl atom: . During the rotation, the electron energy will exhibit a Doppler shift , which changes in the interval (− kωR n ,+ kωR n ) due to the change in the angle between v n and the electron momentum k . This variation of the Doppler shift results in a Doppler line broadening which is different for light ( n =H) and heavy ( n =Cl) atoms. Taking into account that j n = R n × k , we can conclude that the Doppler shift k · v n is nothing else but the rotational Doppler shift j n · ω , which is larger for the light atom. The X-ray polarization vector e is parallel to the electron momentum k , while the photon propagation axis is perpendicular to the figure plane. Full size image Experimental and theoretical rotational envelopes The key results of our investigation are shown in Figs 2 and 3 . Our experimental data (shown by empty circles in Fig. 2 ) clearly confirm the theoretical prediction by Sun et al. [22] As shown in Fig. 2 for v=3, the spectral profile of a single vibrational sub-state following the photoionization of the 5σ electrons of HCl consists of a narrow peak assigned to the ejection of an electron from the Cl site (blue curve) and a broad pedestal related to the emission from the hydrogen atom (black curve) [22] . The analysis of the ‘partial’ H contribution necessitates the subtraction of the Cl contribution from the total spectrum. To extract the broad pedestal from the total spectrum, we took into account that the excitation of the rotational levels composing the Cl peak is due to the transfer of the photon spin S =1 to the molecule. Thus, the Cl profile was simulated using the rotational distribution for the P and R branches extracted from the low-energy photoelectron spectra of Edwardsson et al. [26] as shown in Fig. 2 . The subtraction of the Cl profile with a full width at half maximum (FWHM) of 32 meV (which includes the rotational broadening, the translational Doppler and the instrumental broadenings) results in an ‘experimental profile of the H band’ shown in Fig. 3 by crosses. The simulation of the H profiles corresponding to v=0, ⋯ , 6 was performed by modifying the semi-classical theory of the rotational Doppler and recoil effects [22] , [25] as outlined in the Methods section. The theoretical simulations took into account both the translational Doppler broadening (FWHM=18.8 meV) and the instrumental broadening (FWHM=18 meV), and the result is in good agreement with our experimental data ( Fig. 3 ). The observed asymmetry is caused by the dependence of the rotational recoil shift j 2 ( θ )/2 I on the angle between k and the molecular axis R . 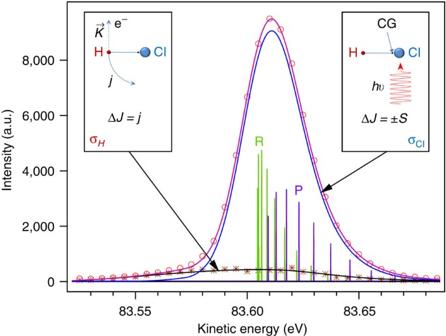Figure 2: Formation of the rotational envelope. The rotational envelope of thev=3 vibrational sub-state (seeFig. 3) consists of a narrow Cl contribution (blue solid line) and a broad pedestal related to the H contribution (black solid line). The Cl contribution is formed by the P and R rotational branches related to the angular momentum transfer from the X-ray photon to the molecule, while the broad H band is mainly due to the angular momentum transfer from the fast photoelectron ejected from the hydrogen atom to the molecule. Figure 2: Formation of the rotational envelope. The rotational envelope of the v =3 vibrational sub-state (see Fig. 3 ) consists of a narrow Cl contribution (blue solid line) and a broad pedestal related to the H contribution (black solid line). The Cl contribution is formed by the P and R rotational branches related to the angular momentum transfer from the X-ray photon to the molecule, while the broad H band is mainly due to the angular momentum transfer from the fast photoelectron ejected from the hydrogen atom to the molecule. 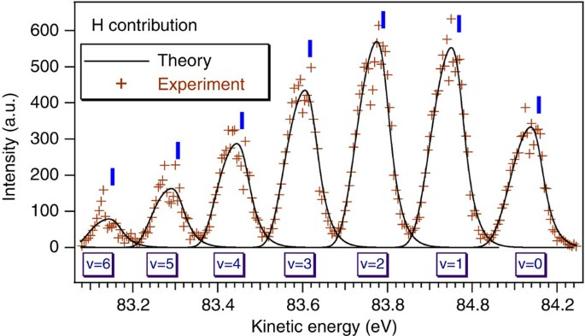Figure 3:Vibrationally resolved photoionization spectrum of HCl for the5σstate. The spectrum was recorded athν=100 eV corresponding to an electron kinetic energyE≈84 eV. Seven vibrational sub-states (v=0,⋯,6) are observed. The experimental (brown crosses) and theoretical (black solid line) partial photoionization spectra correspond to the electron emission from the hydrogen atom (see text). Owing to the rotational recoil effect related to the electron ejection from the hydrogen atom, the broad H peaks are shifted compared with the narrower Cl peaks whose maxima are shown by blue bars. Full size image Figure 3: Vibrationally resolved photoionization spectrum of HCl for the 5σ state. The spectrum was recorded at hν =100 eV corresponding to an electron kinetic energy E ≈84 eV. Seven vibrational sub-states (v=0, ⋯ ,6) are observed. The experimental (brown crosses) and theoretical (black solid line) partial photoionization spectra correspond to the electron emission from the hydrogen atom (see text). Owing to the rotational recoil effect related to the electron ejection from the hydrogen atom, the broad H peaks are shifted compared with the narrower Cl peaks whose maxima are shown by blue bars. Full size image In the same manner as an ice skater spins faster or slower by retracting or extending his arms, structural changes of a molecule change its rotational motion. Both the simulations and the experiment show a narrowing of the H profile (FWHM=88 meV and 83 meV) on the way from v=0 to v=6. The reason is the increase in the moment of inertia for larger v due to the elongation of the effective bond length for higher vibrational sub-states. This structural change, characterized by the parameter β =( I – I f )/ I f , modifies qualitatively the dependence of the electron kinetic energy E on the angular velocity of the molecule ω . Here, I f is the moment of inertia in the final vibrational state. This dispersion law, which is described in detail in the Methods section, is at the origin of the spectral profile of the vibrational sub-states, and changes from a plane for β =0 ( Fig. 4a ) to a paraboloid when β ≠0 ( Fig. 4b ). The best agreement with the experimental data was obtained for the following parameters: β =−0.297, −0.334, −0.361, −0.387, −0.419, −0.446, −0.468, corresponding to the vibrational sub-states v=0, 1, 2, 3, 4, 5, 6, respectively. These β values are in perfect agreement with previous low-energy electron spectroscopy measurements [26] . The site selectivity achieved in photoionization will be magnified by the increase of the photon energy due to a dramatic enlargement of both rotational broadening D and rotational shift Δ (see Fig. 4c ). 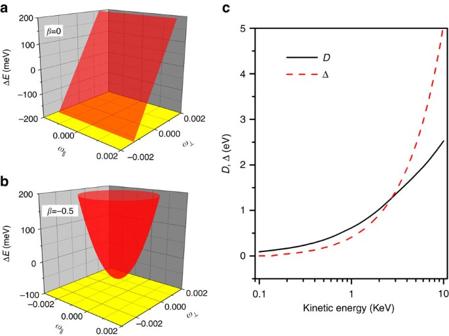Figure 4:Dispersion law ΔE=ΔE(ω). It describes the dependence of the electron energy on the angular velocityin the ground state, whereand, respectively ,are the parallel and the perpendicular components ofωwith respect to the recoil angular momentumj=[RH×k]. This dispersion law, responsible for the formation of the rotational envelope of the individual vibrational sub-states (see Methods section), is very sensitive to the change in the moment of inertia during photoionization. It is qualitatively different for (a)β=0 and for (b)β≠0 (see text). The position of the bottom of the paraboloid is (ΔE=−42 meV,,) forβ=−0.5, while the position of the top of the paraboloid is (ΔE=124 meV,,) forβ=0.5. (c) Rotational Doppler broadeningD(FWHM), and shift Δ, caused by the rotational recoil effect, computed as the width and shift of the spectrum (1) for the hydrogen atom in room temperature (T=300 K) HCl. Figure 4: Dispersion law Δ E =Δ E ( ω ). It describes the dependence of the electron energy on the angular velocity in the ground state, where and , respectively ,are the parallel and the perpendicular components of ω with respect to the recoil angular momentum j =[ R H × k ]. This dispersion law, responsible for the formation of the rotational envelope of the individual vibrational sub-states (see Methods section), is very sensitive to the change in the moment of inertia during photoionization. It is qualitatively different for ( a ) β =0 and for ( b ) β ≠0 (see text). The position of the bottom of the paraboloid is (Δ E =−42 meV, , ) for β =−0.5, while the position of the top of the paraboloid is (Δ E =124 meV, , ) for β =0.5. ( c ) Rotational Doppler broadening D (FWHM), and shift Δ, caused by the rotational recoil effect, computed as the width and shift of the spectrum (1) for the hydrogen atom in room temperature ( T =300 K) HCl. Full size image Molecular photoionization is often accompanied by geometry changes that can be monitored in various ways, and in particular by photoelectron spectroscopy. In this context, photoelectron spectroscopy with rotational resolution is only achievable at very low photoelectron kinetic energies, and probably one of the most efficient tools to detect small variations in the molecular structure. Indeed, even small changes in the bond distances and angles, or in the atomic masses, alter the rotational spectrum in predictable and measurable ways. However, unlike low-energy valence photoelectron spectroscopy, which is generally not site specific, the significant increase of the photoelectron momentum in X-ray photoionization brings in a new aspect—the separation of overlapping rotational bands according to the ionization site ( Fig. 2 ). Here we report a novel technique, which allows one to give insight into the molecular structure by separating the overlapping rotational bands using the site selectivity of the rotational excitation during X-ray photoionization. The site dependence revealed in this study originates from the fact that the torque, which governs the strength of the rotational excitation and hence the shape of the rotational band, is very different for different atoms in a molecule due to different ‘levers’ and different masses. Thus, it carries MO composition and structural information. The present work clearly demonstrates the important and unique possibility of using the rotational degrees of freedom to unravel the site specificity of molecular valence ionization. Using the textbook case of a hydrogen chloride molecule, we provide a first example of a general phenomenon, namely the site selectivity of the X-ray valence photoionization. We showed that the ejection of a fast photoelectron from light atoms in a molecule gives rise to a broad Doppler pedestal of the spectral profile, which is shifted relative to the narrow peaks corresponding to the emission from the heavy atoms. The present results open the doorway to extensive investigations of site-selective rotational excitation in a wide range of molecules containing light atoms. We would like to suggest at this point that ultrafast [27] pump-probe spectroscopy, which already allowed efficient tracking of nuclear dynamics in molecules [28] , might be a very interesting direction to follow in the future due to its capability to monitor in real time the site-specific coherent rotational motion induced by fast photoelectrons. Experimental methods Experiments have been carried out at the soft X-ray PLEIADES beamline [29] of the SOLEIL synchrotron (France) dedicated to high-resolution spectroscopy [30] , [31] of dilute matter. An 80-mm period Apple II undulator was used, which covers the energy range 35(55)–1,000 eV for a horizontal (vertical) orientation of the polarization vector e . The measurements were performed using a wide-angle lens VG-Scienta R4000 electron spectrometer installed at a fixed position, with the electron detection axis perpendicular to the storage ring plane. X-ray light polarization was set collinear to the electron detection axis . The gas phase sample HCl was provided by Air Liquide with a stated purity better than 99.95%. It was introduced at room temperature in a gas cell with polarized electrodes, which were adjusted to minimize the effect of plasma potentials caused by the ion density gradient created along the synchrotron beam propagating through the gas cell. The gas pressure in the spectrometer vacuum chamber was kept constant at about 6.5 × 10 −6 mbar for all measurements. The total instrumental broadening for a photoelectron kinetic energy E ≈84 eV was FWHM=18 meV, while the translational Doppler broadening was FWHM=18.8 meV. A Pt-coated diffraction grating with 1,600 lines per mm was used to produce monochromatic X-rays with the photon energy hν =100 eV, corresponding to a photoelectron kinetic energy of E ≈84 eV. Theoretical methods The spectral shape of a single vibrational sub-state in X-ray photoionization, involving the rotational structure, was computed by modifying the semi-classical approach established in ref. 22 and taking into account the elongation of the bond length when increasing the vibrational quantum number ν where Θ[ x ] is the step function and Δ E ≡ E −( hν − I 5 σ ), , j (θ)= kR ( m Cl / M ) sin θ , , Δ 0 ( θ )=Δ E + j 2 ( θ )/2 I + k 2 /2 M , M = m H + m Cl is the total mass of the molecule, k B is the Boltzmann constant. The change in the moment of inertia β =( I − I f )/ I f modifies the Doppler shift . The rotational recoil results in a shift j 2 ( θ )/2 I , as well as in an additional broadening caused by the angular dependence of the recoil angular momentum j ( θ ). We would like to point out that in equation (1), we neglect the scattering of the outgoing electron wave by the neighbouring atom. Our analysis indicates that this scattering contribution is very small and does not influence the rotational profile within our experimental accuracy. To make possible a comparison with the experimental data, the spectrum (1) σ(Δ E − ε ) was convoluted with a Gaussian exp(−4ε 2 ln2/ γ 2 ), where γ =FWHM=26 meV includes the total instrumental and translational Doppler broadenings. The rotational profile (1) differs qualitatively from the conventional one [22] , because the change in the moment of inertia drastically modifies the dispersion law where z =− j 2 ( θ )/2 I − k 2 /2 M . Since β ≠0, the dispersion law deviates from for β =0 (see Fig. 4 ). This effect resembles the Fortrat effect [32] for the photon-induced rotational excitation Δ J =±1. How to cite this article: Miron, C. et al. Site-selective photoemission from delocalized valence shells induced by molecular rotation. Nat. Commun. 5:3816 doi: 10.1038/ncomms4816 (2014).